Bacterial Pili exploit integrin machinery to promote immune activation and efficient blood-brain barrier penetration Group B Streptococcus (GBS) is the leading cause of meningitis in newborn infants. Bacterial cell surface appendages, known as pili, have been recently described in streptococcal pathogens, including GBS. The pilus tip adhesin, PilA, contributes to GBS adherence to blood-brain barrier (BBB) endothelium; however, the host receptor and the contribution of PilA in central nervous system (CNS) disease pathogenesis are unknown. Here we show that PilA binds collagen, which promotes GBS interaction with the α 2 β 1 integrin resulting in activation of host chemokine expression and neutrophil recruitment during infection. Mice infected with the PilA-deficient mutant exhibit delayed mortality, a decrease in neutrophil infiltration and bacterial CNS dissemination. We find that PilA-mediated virulence is dependent on neutrophil influx as neutrophil depletion results in a decrease in BBB permeability and GBS–BBB penetration. Our results suggest that the bacterial pilus, specifically the PilA adhesin, has a dual role in immune activation and bacterial entry into the CNS. Bacterial meningitis, a serious infection of the central nervous system (CNS), is a major cause of death and disability worldwide. Streptococcus agalactiae (Group B Streptococcus , GBS), a Gram-positive bacterial pathogen, is the leading cause of meningitis in human newborns, and increasingly associated with invasive disease in the elderly. Despite the introduction of intrapartum antibiotic prophylaxis in pregnant women to prevent GBS transmission, mortality rates in neonates remain high (10%), and 25–50% of surviving infants experience permanent neurologic sequelae, including cerebral palsy, seizure activity, deafness and/or blindness [1] . Brain damage following GBS meningitis likely results from the loss of blood-brain barrier (BBB) integrity due to toxicity of bacterial products and/or activation of host inflammatory mediators that compromise BBB function [2] . The human BBB, which is mainly composed of a single layer of specialized human brain microvascular endothelial cells (hBMEC), serves as a critical barrier to protect the CNS against microbial invasion. It is postulated that GBS interaction with hBMEC, is the primary step in the pathogenesis of meningitis, whereon a combination of bacterial transcytosis, endothelial cell injury, and inflammatory mechanisms combine to disrupt the BBB [3] . Cell surface organelles called pili were recently discovered in GBS and other streptococcal pathogens [4] , [5] , [6] . Pili are flexible appendages on the bacterial surface that have been shown to participate in essential events for infection establishment, including adhesion to the host cells, DNA transfer and biofilm formation [7] . Pili in Gram-positive bacteria consist of a backbone formed by covalently linked monomers of a major pilin with associated minor pilin proteins that have been shown to be essential for adhesion to a variety of host tissues [8] , [9] , [10] . The genes encoding pili in GBS are located within two distinct loci, designated as pilus island 1 and 2 (PI-1 and PI-2), with two variants of PI-2: PI-2a and PI-2b [11] . The overall gene organization of the two islands is similar that consists of three genes that encode LPXTG motif-carrying proteins corresponding to the major pilus subunit (PilB), two ancillary proteins (PilA and PilC) along with two genes encoding transpeptidase enzymes (sortases) involved in pilus assembly [12] . All clinical isolates of GBS carry at least one of the two pilus islands [13] . We have demonstrated previously that GBS clinical isolate NCTC10/84 (serotype V) expresses pili and that the pilus adhesin, PilA, contributes to GBS adherence to brain endothelium [8] . However, the identity of the host cell receptor and the contribution of GBS pili to the pathogenesis of CNS disease are largely unknown. In this study, we examine the global gene expression profile of brain endothelium to infection with a GBS isogenic Δ pilA mutant using microarray, real-time PCR with reverse transcription (RT–PCR), and protein analysis. Our studies suggest that BBB endothelium responds to the GBS PilA with functional gene expression to promote the characteristic neutrophilic inflammatory response of acute bacterial meningitis. We also demonstrate that PilA interacts directly with collagen to engage integrins and integrin signalling machinery, which contributes to the pathogenesis of meningitis in vivo . GBS PilA induces chemokine expression in brain endothelium We have previously demonstrated that BBB endothelium has an active role in initiating a specific innate immune response to GBS infection, promoting neutrophil activation and recruitment [3] , [14] . In this study, global transcriptional analysis of hBMEC during infection with a GBS PilA-deficient mutant revealed a marked reduction in the expression of CXC family of neutrophil chemokines IL-8, CXCL-1, and CXCL-2, as well as CCL-20 and IL-6, compared to infection with WT GBS ( Supplementary Table S1 ). These results were confirmed in independent experiments using real-time RT–PCR ( Fig. 1a ), further suggesting that the hBMEC transcriptional response is influenced by a PilA-mediated interaction. 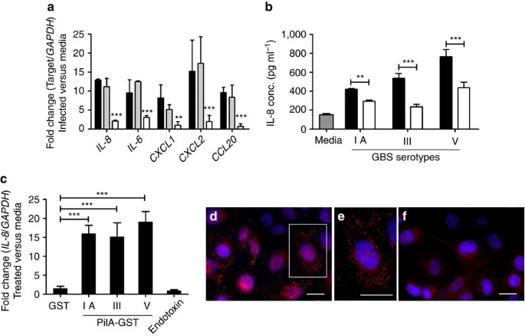Figure 1: PilA promotes chemokine induction in brain endothelium. (a) Real-time RT–PCR analysis of chemokines IL-8, IL-6, CXCL1, CXCL2 and CCL20 in hBMEC 4 h post infection with WT GBS (black bars) or isogenic mutants Δsrr-1(grey bars) and ΔpilA(white bars). Transcript levels were normalized to GAPDH and fold change was determined as described in Methods; statistical analysis was performed with two-way ANOVA (Bonferroni test). (b) IL-8 secretion by hBMEC on infection with GBS WT strains (black bars) and isogenic ΔpilAmutants (white bars). Concentrations of IL-8 in hBMEC supernatants collected 4 h post infection were measured using ELISA, two-way ANOVA (Bonferroni test); **P<0.005; ***P<0.001. (c) Transcript levels of IL-8 following treatment (4 h) with PilA–GST fusion proteins from different GBS serotypes as well as control GST protein (0.5 μM) andE. coliendotoxin (0.3 ng ml−1). Cells were treated with the amount of endotoxin that were detected in PilA–GST fusion proteins and GST control protein preparations with a endotoxin detection kit, as described in Methods; statistical analysis with one-way ANOVA (Tukey's multiple comparison test). All experiments were performed three times in triplicate wells, and bars represent the standard deviation of the mean of one representative experiment, **P<0.005; ***P<0.001. (d–f) Binding of purified PilA–GST protein to hBMEC. Cells were treated with PilA–GST (d) or GST (f) and then probed with either Anti-PilA antiserum or Anti-GST Ab. Nucleus is stained with DAPI. Magnification of the boxed area in 'd' is shown in 'e'. Scale bar, 20 μm. Figure 1: PilA promotes chemokine induction in brain endothelium. ( a ) Real-time RT–PCR analysis of chemokines IL-8, IL-6, CXCL1, CXCL2 and CCL20 in hBMEC 4 h post infection with WT GBS (black bars) or isogenic mutants Δ srr-1 (grey bars) and Δ pilA (white bars). Transcript levels were normalized to GAPDH and fold change was determined as described in Methods; statistical analysis was performed with two-way ANOVA (Bonferroni test). ( b ) IL-8 secretion by hBMEC on infection with GBS WT strains (black bars) and isogenic Δ pilA mutants (white bars). Concentrations of IL-8 in hBMEC supernatants collected 4 h post infection were measured using ELISA, two-way ANOVA (Bonferroni test); ** P <0.005; *** P <0.001. ( c ) Transcript levels of IL-8 following treatment (4 h) with PilA–GST fusion proteins from different GBS serotypes as well as control GST protein (0.5 μM) and E. coli endotoxin (0.3 ng ml −1 ). Cells were treated with the amount of endotoxin that were detected in PilA–GST fusion proteins and GST control protein preparations with a endotoxin detection kit, as described in Methods; statistical analysis with one-way ANOVA (Tukey's multiple comparison test). All experiments were performed three times in triplicate wells, and bars represent the standard deviation of the mean of one representative experiment, ** P <0.005; *** P <0.001. ( d – f ) Binding of purified PilA–GST protein to hBMEC. Cells were treated with PilA–GST ( d ) or GST ( f ) and then probed with either Anti-PilA antiserum or Anti-GST Ab. Nucleus is stained with DAPI. Magnification of the boxed area in ' d ' is shown in ' e '. Scale bar, 20 μm. Full size image The pilA gene encoded in PI-2a and is highly homologous between GBS strains that harbour this locus (~89% identity). To investigate the role of PilA proteins in other GBS serotypes commonly associated with GBS meningitis, we constructed pilA targeted mutants in GBS strains NEM316 (serotype III) and 515 (serotype 1a) ( Supplementary Fig. S1a ). No difference in the growth kinetics or hemolytic activity was observed between the respective WT and Δ pilA mutant strains ( Supplementary Fig. S1b,c ). Consistent with our microarray analysis, infection with the PilA-deficient strains resulted in less IL-8 protein secretion compared with the respective WT parental strains ( Fig. 1b ). Complementation of the Δ pilA mutant with the intact pilA gene restored hBMEC IL-8 secretion to that observed during infection with WT GBS ( Supplementary Fig. S1d ). PilA promotes IL-8 secretion and neutrophil chemotaxis We next sought to determine whether GBS PilA is sufficient to induce IL-8 using purified recombinant PilA. PilA proteins, from several serotype strains, were expressed as amino-terminal GST tagged fusion proteins ( Supplementary Fig. S2a ). Following purification, all proteins, including the GST protein control, contained low endotoxin levels (3 EU ml −1 or 0.3 ng ml −1 ). Treatment of hBMEC with PilA–GST proteins resulted in a significant induction of IL-8 transcription ( Fig. 1c ). We also observed direct PilA protein binding to hBMEC compared with that of the GST control protein ( Fig. 1d–f ). We further analysed neutrophil recruitment to the site of infection using a cutaneous in vivo neutrophil recruitment assay, as described previously [15] . Neutrophil enzyme myeloperoxidase (MPO), which serves as an effective indicator of neutrophil infiltration [16] , was significantly lower after infection with the Δ pilA mutant compared with the WT strain ( Fig. 2a ). This increased neutrophil recruitment was independent of the number of bacteria present in the tissue, as similar bacterial colony-forming units (CFU) were recovered from the skin for both the WT and Δ pilA mutant under these conditions ( Fig. 2b ). Similar results were observed when assessing polymorphornuclear (PMN) cell recruitment directly in the CNS. Mice injected intracranially with the Δ pilA mutant exhibited less PMN infiltrate compared with animals inoculated with WT GBS ( Fig. 2c–h ). Taken together, these results indicate that GBS PilA promotes IL-8 secretion and functional neutrophil signalling pathways in vivo , resulting in neutrophil recruitment during active GBS infection. 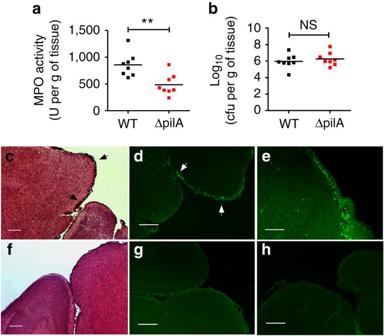Figure 2: PilA induces neutrophil chemotaxis. (a)In vivoneutrophil recruitment was assessed by measuring MPO activity in mice (CD1, male,n=8 per group) skin homogenates 4 h post infection either with WT GBS (black squares) or ΔpilAmutant (red squares). MPO assays were performed on mice skin homogenates after subcutaneous injection with 1×106CFU of either WT GBS or ΔpilAmutant strain. (b) Bacterial counts in skin homogenates were assessed by plating serial-fold dilutions on Todd-Hewitt broth agar plates. Experiments were performed twice, a representative experiment is shown. Bars represent mean MPO levels or bacterial cfu, statistical analaysis was performed using Student'st-test; **P<0.005; NS, non-significant. (c–h) Neutrophil recruitment in the CNS was assessed following direct intracranial injection in 5-day-old mice (n=4 per group) 8–10 h post inoculation with WT GBS or ΔpilAmutant. Representative images of brains from two independent experiments are shown for two mice (c–e) infected with WT (same mouse inc,d) and two mice (f–h) infected with ΔpilAmutant (same mouse inf,g). Brain sections stained with hematoxylin and eosin (H&E) (c,f) depict meningeal thickening during WT infection (c, arrows) and PMN infiltration by immunohistochemical detection with FITC–anti-Ly6G Ab (d,e,g,h). Scale bar, 20 μm. Figure 2: PilA induces neutrophil chemotaxis. ( a ) In vivo neutrophil recruitment was assessed by measuring MPO activity in mice (CD1, male, n =8 per group) skin homogenates 4 h post infection either with WT GBS (black squares) or Δ pilA mutant (red squares). MPO assays were performed on mice skin homogenates after subcutaneous injection with 1×10 6 CFU of either WT GBS or Δ pilA mutant strain. ( b ) Bacterial counts in skin homogenates were assessed by plating serial-fold dilutions on Todd-Hewitt broth agar plates. Experiments were performed twice, a representative experiment is shown. Bars represent mean MPO levels or bacterial cfu, statistical analaysis was performed using Student's t -test; ** P <0.005; NS, non-significant. ( c – h ) Neutrophil recruitment in the CNS was assessed following direct intracranial injection in 5-day-old mice ( n =4 per group) 8–10 h post inoculation with WT GBS or Δ pilA mutant. Representative images of brains from two independent experiments are shown for two mice ( c – e ) infected with WT (same mouse in c , d ) and two mice ( f – h ) infected with Δ pilA mutant (same mouse in f , g ). Brain sections stained with hematoxylin and eosin (H&E) ( c , f ) depict meningeal thickening during WT infection ( c , arrows) and PMN infiltration by immunohistochemical detection with FITC–anti-Ly6G Ab ( d , e , g , h ). Scale bar, 20 μm. Full size image Collagen promotes PilA–BBB interaction Sequence analysis of GBS PilA as well as comparison to a recent crystal structure of a GBS PilA orthologue [17] reveals several distinct domains including two Cna-B-like domains, which are similar to IgG domains found in S. aureus adhesins [18] , and an Integrin I-like domain that resembles the A3 domain of human von Willebrand factor, a molecule shown to interact with collagens [19] . Because a recent report demonstrated that the PilA von Willebrand factor region confers adherent properties to host cells [20] , we further hypothesized that this may include PilA-mediated binding to collagen. We first observed that binding to immobilized collagen I was impaired in the Δ pilA mutant ( Fig. 3a ). Direct binding of purified PilA–GST protein to collagen I was also assessed in an enzyme-linked immunosorbent (ELISA)-based assay where we observed a dose-dependent increase in the binding of the PilA protein, and not the GST control, to collagen ( Fig. 3b ). When GBS was incubated with increasing amounts of collagen, we observed an increase in both bacterial attachment and internalization of WT GBS and not the Δ pilA mutant strain ( Fig. 3c, d ; Supplementary Fig. S2b,c ). Further, PilA-coated latex beads bound hBMEC more abundantly in the presence of collagen compared with BSA or GST-coated beads ( Fig. 3e ). These results suggest that collagen promotes PilA–hBMEC interaction. 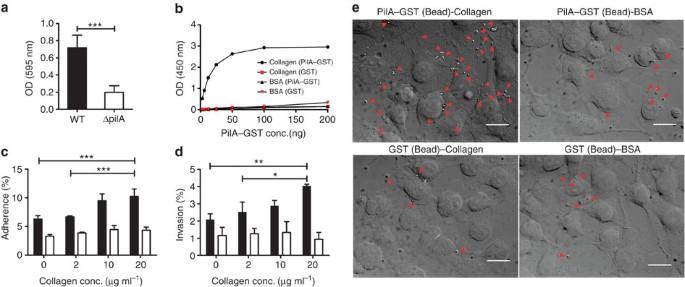Figure 3: PilA binds to collagen. (a) Binding of WT GBS and ΔpilAmutant to immobilized collagen was assessed by crystal violet staining. Stain released from attached bacteria was quantified by measuring absorbance at 595 nm. Student'st-test. (b) Dose-dependent binding of recombinant PilA protein to collagen I or BSA compared with GST control protein was measured by ELISA as described in Methods. Adherence (c) and invasion (d) of WT GBS (black bars) and ΔpilAmutant (white bars) in the presence increasing amount of collagen I. Bacteria were preincubated with indicated concentration of soluble collagen, washed extensively and assayed for the ability to adhere and invade the hBMEC by antibiotic protection assay. Data are reported as percent adherent or intracellular bacteria relative to the inuput inoculum. All experiments were performed three times in triplicate and bars represent means and standard deviations of one representative experiment. Statistical analysis was performed using Student'st-test (a) or one-way ANOVA with Tukey's multiple comparison test (all other experiments) (*P<0.05; **P<0.005; ***P<0.001. (e) Phase contrast images of PilA–GST, GST or BSA-coated latex beads binding to hBMEC in the presence of collagen or BSA. Cells were extensively washed with PBS to remove any unbound or loosely bound beads and visualized using a Zeiss Axiovert 200 inverted microscope (Carl Zeiss). Arrows indicate beads on hBMEC surface. Scale bar, 20 μm. Figure 3: PilA binds to collagen. ( a ) Binding of WT GBS and Δ pilA mutant to immobilized collagen was assessed by crystal violet staining. Stain released from attached bacteria was quantified by measuring absorbance at 595 nm. Student's t -test. ( b ) Dose-dependent binding of recombinant PilA protein to collagen I or BSA compared with GST control protein was measured by ELISA as described in Methods. Adherence ( c ) and invasion ( d ) of WT GBS (black bars) and Δ pilA mutant (white bars) in the presence increasing amount of collagen I. Bacteria were preincubated with indicated concentration of soluble collagen, washed extensively and assayed for the ability to adhere and invade the hBMEC by antibiotic protection assay. Data are reported as percent adherent or intracellular bacteria relative to the inuput inoculum. All experiments were performed three times in triplicate and bars represent means and standard deviations of one representative experiment. Statistical analysis was performed using Student's t -test ( a ) or one-way ANOVA with Tukey's multiple comparison test (all other experiments) (* P <0.05; ** P <0.005; *** P <0.001. ( e ) Phase contrast images of PilA–GST, GST or BSA-coated latex beads binding to hBMEC in the presence of collagen or BSA. Cells were extensively washed with PBS to remove any unbound or loosely bound beads and visualized using a Zeiss Axiovert 200 inverted microscope (Carl Zeiss). Arrows indicate beads on hBMEC surface. Scale bar, 20 μm. Full size image Role of α 2 β 1 integrin and FAK signalling in BBB activation Extracellular matrix proteins like collagen typically interact with cell surface integrins to initiate downstream signalling cascades mediated through Focal adhesion kinase (FAK), which is central to integrin-mediated signalling [21] . 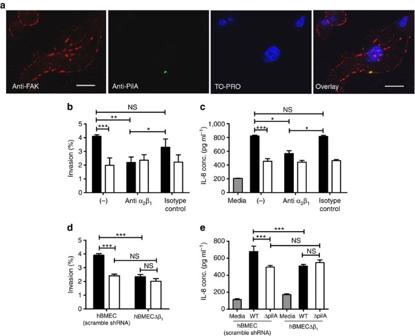Figure 4: PilA interacts with α2β1integrins to promote bacterial penetration and chemokine secretion. (a) Co-localization of PilA-coated latex beads with FAK visualized by confocal microscopy. PilA-coated beads are stained with Anti-PilA antiserum (green), FAK with Anti-FAK monoclonal Ab (red) and nucleus with To-Pro (blue). Scale bar, 100 μm. Inhibition of GBS internalization (b) and IL-8 secretion (c) by hBMEC following pretreatment with α2β1integrin function blocking monoclonal Ab compared with isotype control Ab. GBS penetration (d) and IL-8 release (e) in β1integrin knockdown hBMEC cells using shRNA targeting β1integrin RNA (hBMEC Δβ1) or a control shRNA (scramble shRNA). Bacterial invasion was quantified by antibiotic protection assay and IL-8 secretion was measured by ELISA. Black bars represent WT GBS and white bars represent ΔpilAmutant. All experiments were performed three times in triplicate and bars represent the standard deviation of the mean of one representative experiment. Statistical analysis was performed using one-way ANOVA (Tukey's multiple comparison test); *P<0.05; **P<0.005; ***P<0.001; NS, non-significant. As shown in Figure 4a , confocal microscopy depicted co-localization of PilA–GST-coated latex beads with FAK at the focal adhesion sites. This led us to investigate whether integrins, which are present in focal adhesion sites, might be acting as the host receptor for PilA. Cells generally express two predominantly collagen binding integrins: α 1 β 1 and α 2 β 1 (ref. 22 ). Previous integrin profiling studies revealed that hBMEC only express α 2 and β 1 integrins [23] . When α 2 β 1 or β 1 integrins were blocked using respective function-blocking monoclonal antibodies, we observed a significant reduction in WT GBS attachment and invasion in hBMEC compared with an isotype control antibody ( Fig. 4b ; Supplementary Fig. S3a,b ). There was no noteworthy change in the adherence and invasive capabilities of the Δ pilA mutant strain, indicating that α 2 β 1 integrins are required for PilA-mediated GBS penetration of BBB endothelium. Interestingly, IL-8 secretion by hBMEC on infection with WT GBS was also significantly reduced in presence of both α 2 β 1 or β 1 integrin function-blocking monoclonal antibodies ( Fig. 4c ; Supplementary Fig. S3c ). Furthermore, as described in the Methods, we knocked down the expression of β 1 integrin in hBMEC by short hairpin RNA ( Supplementary Fig. S3d ). Bacterial invasion, as well as IL-8 secretion on infection with WT GBS, was significantly reduced in β 1 integrin knockdown hBMEC cells compared with cells transfected with the scramble shRNA control ( Fig. 4d,e ). Finally, we observed a significant reduction in PilA–GST binding to β 1 integrin knockdown hBMEC cells, as well as in cells treated with anti-α 2 β 1 monoclonal Ab, as compared with cells transfected with the scramble shRNA control ( Supplementary Fig. S3e–g ). These results further suggest that integrin α 2 β 1 acts as a receptor for GBS PilA. Figure 4: PilA interacts with α 2 β 1 integrins to promote bacterial penetration and chemokine secretion. ( a ) Co-localization of PilA-coated latex beads with FAK visualized by confocal microscopy. PilA-coated beads are stained with Anti-PilA antiserum (green), FAK with Anti-FAK monoclonal Ab (red) and nucleus with To-Pro (blue). Scale bar, 100 μm. Inhibition of GBS internalization ( b ) and IL-8 secretion ( c ) by hBMEC following pretreatment with α 2 β 1 integrin function blocking monoclonal Ab compared with isotype control Ab. GBS penetration ( d ) and IL-8 release ( e ) in β 1 integrin knockdown hBMEC cells using shRNA targeting β 1 integrin RNA (hBMEC Δβ 1 ) or a control shRNA (scramble shRNA). Bacterial invasion was quantified by antibiotic protection assay and IL-8 secretion was measured by ELISA. Black bars represent WT GBS and white bars represent Δ pilA mutant. All experiments were performed three times in triplicate and bars represent the standard deviation of the mean of one representative experiment. Statistical analysis was performed using one-way ANOVA (Tukey's multiple comparison test); * P <0.05; ** P <0.005; *** P <0.001; NS, non-significant. Full size image The non-receptor FAK localizes with β 1 integrins and becomes activated in response to integrin initiated signalling processes [21] . Previously, phosphorylation of FAK was shown to be crucial for invasion of hBMEC by a GBS serotype III strain [24] . We similarly show that FAK, as well as Akt and Erk1/2, are phosphorylated during WT GBS infection, whereas little-to-no phosphorylation was observed during infection with the Δ pilA mutant over the same time period ( Fig. 5a ). To further examine the impact of FAK on PilA-mediated cellular invasion and IL-8 secretion, hBMECs were transfected with the carboxy-terminally truncated FAK-derivative FRNK (FAK-related non-kinase), which does not contain an active kinase domain, and acts as a dominant negative form when overexpressed in hBMEC (FRNK/hBMEC) [25] . 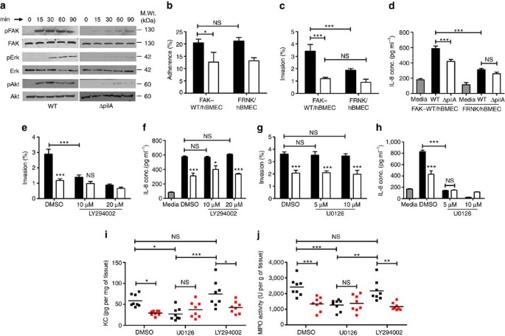Figure 5: FAK is central to GBS invasion and chemokine secretion. (a) Detection of phosphorylated forms of FAK (Tyr-397), Akt (Ser-473) and Erk1/2 (Tyr-204) as well as non-phosphorylated forms in hBMEC lysates at different stages of infection with WT GBS and ΔpilAmutant. Cells were infected for indicated time points, and cell lysates collected were probed with respective antibodies. Adherence (b), Invasion (c) and IL-8 secretion from (d) FRNK/hBMEC compared with FAK–WT/hBMEC on infection with WT GBS (black bars) or ΔpilAmutant (white bars). hBMECs were transfected with the C-terminally truncated FAK derivative FRNK (FAK-related non-kinase), which acts as a dominant negative form when overexpressed (FRNK/hBMEC). Bacterial invasion (e,g) and IL-8 secretion in hBMEC (f,h) on infection with WT GBS (black bars) or ΔpilAmutant (white bars) in presence of PI3K inhibitor LY294002 (e,f) or MEK1/2 inhibitor U0126 (g,h). All experiments were performed three times in triplicate and bars represent the standard deviation of the mean. Statistical analysis was performed using one-way ANOVA (Tukey's multiple comparison test); *P<0.05; ***P<0.001; ns: non-significant. KC levels (i) and MPO activity (j) in mice (n=8 per group) skin homogenates 4 h post subcutaneous injection with either WT GBS (black squares) or ΔpilAmutant (red squares). 2 h before bacterial injection mice were injected subcutaneously with 1 mg kg−1of either U0126, LY294002 or DMSO as a control. Experiments were performed twice and bars represent means and standard deviations of one representative experiment. All experiments were analysed by one-way ANOVA (Tukey's multiple comparison test); *P<0.05; **P<0.005; ***P<0.001; NS, non significant. We did not observe any change in bacterial adherence between different cell lines during infection with either WT GBS or Δ pilA mutant ( Fig 5b ). However, we did observe a reduction in cellular invasion and IL-8 secretion during WT GBS infection of FRNK/hBMEC cells compared with the WT FAK control ( Fig. 5c,d ). To examine whether bacterial invasion itself is required for PilA-mediated IL-8 secretion, we used cytochalasin D to block actin polymerization in hBMEC during GBS infection. This treatment inhibited bacterial internalization in a dose-dependent manner, but did not lead to a reduction in bacterial adherence or PilA-mediated IL-8 secretion ( Supplementary Fig. S4 ). Taken together, these results confirm that GBS invasion of brain endothelium is not a prerequisite for IL-8 secretion and imply that PilA mediated engagement of α 2 β 1 integrins initiates FAK signalling events that lead to both chemokine secretion and bacterial penetration. Figure 5: FAK is central to GBS invasion and chemokine secretion. ( a ) Detection of phosphorylated forms of FAK (Tyr-397), Akt (Ser-473) and Erk1/2 (Tyr-204) as well as non-phosphorylated forms in hBMEC lysates at different stages of infection with WT GBS and Δ pilA mutant. Cells were infected for indicated time points, and cell lysates collected were probed with respective antibodies. Adherence ( b ), Invasion ( c ) and IL-8 secretion from ( d ) FRNK/hBMEC compared with FAK–WT/hBMEC on infection with WT GBS (black bars) or Δ pilA mutant (white bars). hBMECs were transfected with the C-terminally truncated FAK derivative FRNK (FAK-related non-kinase), which acts as a dominant negative form when overexpressed (FRNK/hBMEC). Bacterial invasion ( e , g ) and IL-8 secretion in hBMEC ( f , h ) on infection with WT GBS (black bars) or Δ pilA mutant (white bars) in presence of PI3K inhibitor LY294002 ( e , f ) or MEK1/2 inhibitor U0126 ( g , h ). All experiments were performed three times in triplicate and bars represent the standard deviation of the mean. Statistical analysis was performed using one-way ANOVA (Tukey's multiple comparison test); * P <0.05; *** P <0.001; ns: non-significant. KC levels ( i ) and MPO activity ( j ) in mice ( n =8 per group) skin homogenates 4 h post subcutaneous injection with either WT GBS (black squares) or Δ pilA mutant (red squares). 2 h before bacterial injection mice were injected subcutaneously with 1 mg kg −1 of either U0126, LY294002 or DMSO as a control. Experiments were performed twice and bars represent means and standard deviations of one representative experiment. All experiments were analysed by one-way ANOVA (Tukey's multiple comparison test); * P <0.05; ** P <0.005; *** P <0.001; NS, non significant. Full size image We further investigated the role of phosphatidylinositol-3 kinase (PI3K) as well as the MAP kinase Erk1/2 pathway, both of which signal downstream of FAK, during PilA-mediated immune activation and cellular invasion. Inhibition of PI3K activity with LY294002 resulted in a significant reduction in bacterial invasion without affecting IL-8 secretion ( Fig. 5e,f ). In contrast, treatment of cells with Erk1/2 pathway inhibitor U0126, resulted in a drastic decline in IL-8 release (85%) without perturbing the cellular invasion process ( Fig. 5g,h ). We also analysed the effect of these inhibitors on chemokine secretion and neutrophil chemotaxis in vivo by measuring KC (functional murine homologue of IL-8) and MPO levels as described above. Significantly lower levels of KC and subsequent neutrophil recruitment were observed at the site of WT GBS infection with prior treatment of U0126 ( Fig. 5i,j ). No significant difference was observed when similar treatment was carried out with the PI3 K inhibitor LY294002 or during infection with Δ pilA mutant. Overall, these studies suggest that PilA mediated bacterial invasion and induction of chemokine signalling pathways diverge downstream of FAK in possibly independent pathways. PilA contributes to pathogenesis of meningitis in vivo To examine the contribution of PilA to the pathogenesis of GBS CNS infection in vivo , we employed our mouse model of GBS hematogenous meningitis, as described previously [3] , [26] . Mice (8-week, CD-1 male) were intravenously injected with either WT GBS or Δ pilA mutant. All the WT GBS-infected mice died after 54 h whereas it took 148 h for all the Δ pilA mutant-infected mice to succumb to infection. The median survival time of the WT GBS-infected mice was significantly lower compared with Δ pilA mutant-infected mice ( P =0.036, Log Rank test) ( Fig. 6a ). In a similar separate experiment, mice infected with WT GBS or the Δ pilA mutant, were killed after 24 h to assess bacterial dissemination to the brain. The levels of GBS detected in the blood or spleen of each group of mice were essentially identical whereas the bacterial brain load in Δ pilA -infected mice was significantly lower than in mice infected with WT ( Fig. 6b ). Also the CFU recovered from the brain versus the bloodstream was significantly greater in the mice infected with WT compared with the Δ pilA mutant ( Fig. 6c ). RT–PCR analysis revealed that the mice infected with Δ pilA mutant exhibited decreased brain transcript levels of KC, compared with mice infected with WT GBS ( Fig. 6d ). Histopathological analysis of the brain tissue sections from all the animals infected with WT GBS exhibited classical features of meningitis such as meningeal thickening; massive influx of inflammatory cells, especially neutrophils; and substantial haemorrhaging that were rare or absent in animals infected with Δ pilA mutant strain ( Supplementary Fig. S5 ). 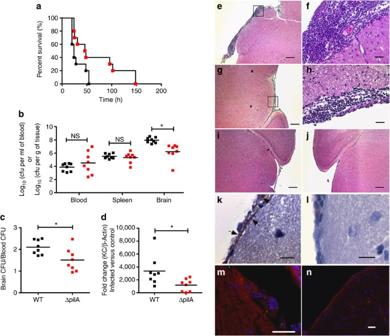Figure 6: Mouse model of GBS meningitis. (a) Kaplan–Meier survival curve of mice following i.v. injection with WT GBS (black sqaures) or ΔpilAmutant (red squares). Groups of CD-1 male mice (n=10 per group) were injected intravenously with 7×107CFU of bacteria and survival was monitored over time and analysed using the Log-rank test; *P<0.05. Bacterial counts in the blood, spleen, brain (cfu per ml or cfu per g of tissue) (b) and ratio of bacterial counts in the brain and blood (c) 24 h post i.v. injection in mice (n=8 per group) with either WT GBS or ΔpilAmutant. (d) Transcript abundance of murine chemokine KC was determined by quantitative RT–PCR on messenger RNA samples isolated from mice brains, following infection with WT GBS or ΔpilAmutant for 24 h. Transcript levels were normalized to β-actin and expressed as fold change compared with mice injected with PBS only. Experiments were performed twice and bars represent standard deviation of the mean of one representative experiment. Statistical analysis was performed using Student'st-test; *P<0.05; NS, non significant. Histopathology of brain tissues of representative individual mice infected with WT GBS (e–h) compared with PBS treatment (i), or infected with ΔpilAmutant (j). Enlargement of boxed areas in 'eandgare shown infandh' respectively, depicting meningeal thickening and neutrophil infiltration. (k–n). Immunohistochemical detection of GBS in the brains of mice infected with either WT GBS (k,m) or ΔpilAmutant (l,n). Bacteria were labelled with monoclonal anti-GBS Ab and detected with anti-mouse secondary antibody conjugated to HRP, coupled with hematoxylin counterstaining (k–l). GBS was also visualized by immunofluorescence with anti-mouse secondary Ab conjugated to AlexaFluor 488 (green). Blood vessels are stained with Anti-laminin Ab (red) and nuclei with To-Pro (blue) (m,n). Scale bar, 20 μm. Images from representative mice infected with WT and the Δ pilA mutant, or following PBS injection, are shown in Figure 6e–j . Presence of WT GBS was visualized in meninges by immunohistochemical analysis, whereas the PilA deficient strain was rarely observed ( Fig. 6k–n ). In a separate experiment, we assessed bacterial load and chemokine expression in multiple tissues, as well as brain pathology during infection with the WT and Δ pilA mutant over time. In general, at all time points tested, even at time of death, mice infected with the Δ pilA mutant had substantially less inflammatory infiltrate and necrotic injury in the brain than those infected with WT GBS ( Supplementary Fig. S6 ). Consistent with our previous experiments, significantly more bacterial CFU and KC expression was observed in the brain and lungs of mice infected with the WT strain ( Supplementary Fig. S7 ). Similar results were obtained in vitro using cervical (HeLa) and lung (A549) epithelial cell lines ( Supplementary Fig. S8 ) demonstrating that PilA contributes to both adherence and chemokine induction in these different cell types. Figure 6: Mouse model of GBS meningitis. ( a ) Kaplan–Meier survival curve of mice following i.v. injection with WT GBS (black sqaures) or Δ pilA mutant (red squares). Groups of CD-1 male mice ( n =10 per group) were injected intravenously with 7×10 7 CFU of bacteria and survival was monitored over time and analysed using the Log-rank test; * P <0.05. Bacterial counts in the blood, spleen, brain (cfu per ml or cfu per g of tissue) ( b ) and ratio of bacterial counts in the brain and blood ( c ) 24 h post i.v. injection in mice ( n =8 per group) with either WT GBS or Δ pilA mutant. ( d ) Transcript abundance of murine chemokine KC was determined by quantitative RT–PCR on messenger RNA samples isolated from mice brains, following infection with WT GBS or Δ pilA mutant for 24 h. Transcript levels were normalized to β-actin and expressed as fold change compared with mice injected with PBS only. Experiments were performed twice and bars represent standard deviation of the mean of one representative experiment. Statistical analysis was performed using Student's t -test; * P <0.05; NS, non significant. Histopathology of brain tissues of representative individual mice infected with WT GBS ( e – h ) compared with PBS treatment ( i ), or infected with Δ pilA mutant ( j ). Enlargement of boxed areas in ' e and g are shown in f and h ' respectively, depicting meningeal thickening and neutrophil infiltration. ( k – n ). Immunohistochemical detection of GBS in the brains of mice infected with either WT GBS ( k , m ) or Δ pilA mutant ( l , n ). Bacteria were labelled with monoclonal anti-GBS Ab and detected with anti-mouse secondary antibody conjugated to HRP, coupled with hematoxylin counterstaining ( k – l ). GBS was also visualized by immunofluorescence with anti-mouse secondary Ab conjugated to AlexaFluor 488 (green). Blood vessels are stained with Anti-laminin Ab (red) and nuclei with To-Pro (blue) ( m , n ). Scale bar, 20 μm. Full size image Role of neutrophils during GBS meningitis Our observation that WT GBS-infected mice had a higher level of chemokine KC as well as significant infiltration of leukocytes, especially neutrophils, led us to investigate the contribution of neutrophils to BBB permeability and the progression of GBS meningitis. Mice were rendered neutropenic using monoclonal antibody RB6–8C5 (ref. 27 ) before intravenous (i.v.) infection with GBS; we observed sustained neutropenia during the course of our experiment ( Supplementary Fig. S9 ). Approximately 45% of the RB6–8C5-treated animals succumbed to death within the first 24 h of infection, probably due to septic shock. This was evidenced by drop in body temperature, higher bacterial load in the blood and lungs, and higher levels of sepsis-related cytokines (IL-1β and IL-6) in serum, spleen and lung in neutropenic mice compared with those treated with isotype control Ab ( Supplementary Fig. S10a–h ). Interestingly, the RB6–8C5-treated mice that survived the initial sepsis lived longer and also exhibited lower bacterial counts in the brain compared with control mice ( Fig. 7a–c ). Following survival of sepsis, the median survival time of neutropenic mice was higher compared with control Ab-treated mice (61 versus 46 h). These results suggest that neutropenia may be conferring a survival advantage during GBS CNS disease. We next sought to examine the permeability of brain endothelium by Evans blue (EB) dye extravasation [28] . Mice were either treated with PBS, RB6–8C5 or isotype control Ab followed by i.v. injection of PBS (for PBS-treated mice) or WT GBS (for Ab-treated mice). Mice were killed 24 h post infection following an i.v. injection with EB (100 μl, 2%, w/v). Brains recovered from mice treated with the isotype control Ab were visibly more blue compared with either RB6–8C5 or PBS-treated non-infected mice ( Fig. 7d ). Significantly higher EB leaching into the brain was quantified in mice treated with control Ab compared with neutropenic mice or PBS-treated mice ( Fig. 7e ). Bacterial load in the brain as well as BBB permeability measured by EB extravasation 24 h post infection with the Δ pilA mutant was similar in mice treated with both the neutrophil depleting and isotype control Ab ( Supplementary Fig. S10i,j ). In a separate experiment, we also assessed BBB permeability using FITC-albumin as a tracer [29] . We similarly observed a generalized leakage from blood vessels within the brain parenchyma during GBS infection in mice that were treated with isotype control Ab compared with animals treated with RB6–8C5 Ab or PBS alone ( Fig. 7f–i ). 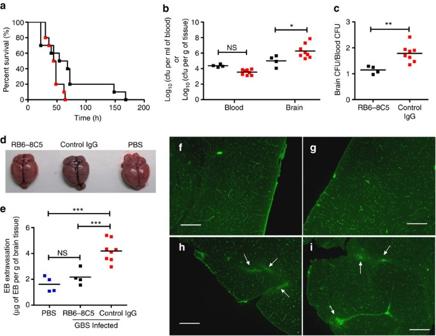Figure 7: Influence of neutropenia on the course of GBS meningitis. (a) Kaplan–Meier survival curve of mice following i.v. injection with 7×107CFU of WT GBS. 24 h before bacterial challenge groups of CD-1 male mice (n=10 per group) were treated intraperitoneally with 50 μg of either neutrophil-depleting Ab, RB6–8C5 (black sqaures) or isotype control Ab (red squares). Survival was monitored at least twice a day over a one-week period and data analysed using Log-rank test;P=0.07. Bacterial counts in the blood, brain (b) and ratio of bacterial counts in the brain versus the blood (c) 24 h post i.v. injection with WT GBS. (d) Pictures of mice brains following i.v. injection of EB dye 1 h before killing. (e) BBB permeability as reflected by amount of EB dye extravasation to the CNS. EB was extracted from brain tissue by treatment with 60% TCA and absorbance was measured at 610 nm. Vascular permeability of the EB dye is expressed as μg of EB per g of brain tissue using a standard curve. Experiments were performed twice and bars represent the standard deviation of the mean of one representative experiment. Statistical analysis was performed using Student'st-test; *P<0.05; **P<0.005; ***P<0.001; NS, non significant. (f–i) Permeability of the BBB as demonstrated by extravasation of FITC–Albumin (10 ml kg−1) that was injected i.v. 30 min before killing. Brains from representative mice are shown following treatment with PBS only (f), infection with WT GBS following treatment with either RB6–8C5 Ab (g) or control IgG (h,i). Arrows indicate areas of dye leakage in the brain. Scale bar, 20 μm. Figure 7: Influence of neutropenia on the course of GBS meningitis. ( a ) Kaplan–Meier survival curve of mice following i.v. injection with 7×10 7 CFU of WT GBS. 24 h before bacterial challenge groups of CD-1 male mice ( n =10 per group) were treated intraperitoneally with 50 μg of either neutrophil-depleting Ab, RB6–8C5 (black sqaures) or isotype control Ab (red squares). Survival was monitored at least twice a day over a one-week period and data analysed using Log-rank test; P =0.07. Bacterial counts in the blood, brain ( b ) and ratio of bacterial counts in the brain versus the blood ( c ) 24 h post i.v. injection with WT GBS. ( d ) Pictures of mice brains following i.v. injection of EB dye 1 h before killing. ( e ) BBB permeability as reflected by amount of EB dye extravasation to the CNS. EB was extracted from brain tissue by treatment with 60% TCA and absorbance was measured at 610 nm. Vascular permeability of the EB dye is expressed as μg of EB per g of brain tissue using a standard curve. Experiments were performed twice and bars represent the standard deviation of the mean of one representative experiment. Statistical analysis was performed using Student's t -test; * P <0.05; ** P <0.005; *** P <0.001; NS, non significant. ( f – i ) Permeability of the BBB as demonstrated by extravasation of FITC–Albumin (10 ml kg −1 ) that was injected i.v. 30 min before killing. Brains from representative mice are shown following treatment with PBS only ( f ), infection with WT GBS following treatment with either RB6–8C5 Ab ( g ) or control IgG ( h , i ). Arrows indicate areas of dye leakage in the brain. Scale bar, 20 μm. Full size image The pathogenesis of GBS meningitis involves haematogenous spread and entry into the CNS by invading the BBB; however, the precise mechanism(s) whereby the bacterium leaves the bloodstream and gains access to the CNS is still being elucidated. In this study, we report that the pilus tip protein, PilA, which mediates GBS attachment to the brain endothelium, contributes to virulence by promoting characteristic neutrophilic infiltrate during acute bacterial meningitis. We further demonstrate that PilA binds the extracellular matrix component collagen, which then engages α 2 β 1 integrins on brain endothelium to dually promote bacterial attachment and proinflammatory chemokine release. Increased neutrophilic infiltrate was correlated with increased BBB permeability and higher levels of bacterial CNS penetration in vivo ( Fig. 8 ). Thus, it is likely that the PilA–BBB interaction represents one of the early molecular events that contribute to disease progression resulting in a detrimental outcome for the host. 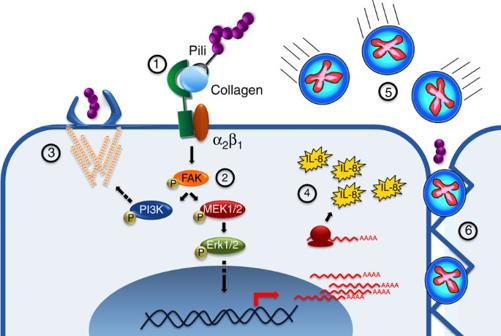Figure 8: Model of GBS PilA-mediated CNS infection. (1) PilA binds the extracellular matrix component collagen, which then engages α2β1integrins on brain endothelium. (2) This leads to FAK activation and subsequent intracellular signalling. (3) Signalling pathway involving PI3K results in actin rearrangement and bacterial uptake. (4) A parallel signalling pathway involving MEK1/2 and Erk1/2 activation leads to IL-8 secretion. (5) This further results in functional neutrophil chemotaxis and activation. (6) Increased neutrophilic infiltrate damages the BBB resulting in increased BBB permeability, which likely facilitates further bacterial passage from the blood stream to the CNS. Figure 8: Model of GBS PilA-mediated CNS infection. (1) PilA binds the extracellular matrix component collagen, which then engages α 2 β 1 integrins on brain endothelium. (2) This leads to FAK activation and subsequent intracellular signalling. (3) Signalling pathway involving PI3K results in actin rearrangement and bacterial uptake. (4) A parallel signalling pathway involving MEK1/2 and Erk1/2 activation leads to IL-8 secretion. (5) This further results in functional neutrophil chemotaxis and activation. (6) Increased neutrophilic infiltrate damages the BBB resulting in increased BBB permeability, which likely facilitates further bacterial passage from the blood stream to the CNS. Full size image The BBB that is primarily composed of a specialized layer of brain microvascular endothelial cells separates the brain and its surrounding tissues maintaining the proper biochemical conditions for normal brain function [30] . Interaction of bacterial components with the BBB is the central event in the pathogenesis of BBB penetration and a prerequisite for development of severe meningeal inflammation, the hallmark of meningitis. GBS factors shown to promote an interaction of the bacterium with brain endothelium include lipotecichoic acid [31] , β-hemolysin/cytolysin (β-h/c) [3] , pili [8] , serine-rich repeat glycoprotein (Srr-1) [26] , fibrinogen-binding protein [32] , laminin-binding protein [33] and recently a hypervirulent GBS adhesin [34] . The majority of these cell surface associated factors directly promote attachment and/or invasion of GBS in different host cell types including hBMEC. We have shown previously that a GBS mutant lacking anchored lipotecichoic acid induced similar levels of IL-8 expression during hBMEC infection as compared with the WT GBS strain [31] . Here we similarly demonstrate that GBS surface adhesin/invasin Srr-1 does not contribute to cytokine/chemokine induction ( Supplementary Table S1 ), suggesting that a reduction in bacterial adherence/invasion is not solely responsible for general decreases in gene transcription observed during infection. We have previously demonstrated that GBS infection of hBMEC results in the upregulation of proinflammatory cytokines and chemokines functioning to orchestrate neutrophil recruitment and activation, and that this effect was largely due to the major cell associated virulence factor β-h/c [3] , [14] . Compared with WT GBS, infection with a PilA-deficient mutant resulted in significantly less gene induction and secretion of key neutrophil CXC chemokines as well as functional neutrophil chemotaxis to the site of infection. We speculate that as pili are long filamentous organelles protruding away from the bacterial surface, pili-mediated contact may represent a crucial first step in GBS–BBB engagement, after which other virulence factors such as the β-h/c toxin will probably contribute to disease progression. Our results that a GBS pilin component contributes to the host proinflammatory response are consistent with recent studies on other piliated pathogens. It was observed that piliated strains of pneumococcus evoked a higher TNFα response than non-piliated strains during systemic infection [5] . Similarly, type I pili (P pili) of uropathogenic Escherichia coli have been shown to stimulate IL-8 release in the urinary tract mucosa [35] . PilA-mediated binding of collagen enhanced GBS attachment as well as uptake into hBMEC in a dose-dependent manner. Our results are consistent with other studies showing that RrgA, the pneumococcal homologue of GBS PilA, binds to various ECM proteins including the collagen [36] , and that minor pilin protein Cpa of Group A Streptococcus (GAS) possess collagen-binding capabilities [37] . The high sequence similarity between RrgA and pilus adhesins from GAS and GBS (identity level of ~50% with similarity levels beyond 70%) points to the possibility that the three-dimensional fold of these proteins could be highly similar, suggesting that pili components may contribute to a general mechanism of pathogen entry and inflammatory induction. Many pathogenic bacteria exploit integrin-mediated signalling for entry into the host cells [38] , [39] . Here we demonstrate that the interaction between PilA and α 2 β 1 integrin in BBB endothelium probably results in FAK activation to initiate signalling pathways leading to both bacterial internalization and proinflammatory cytokine release, which results in functional neutrophil chemotaxis and disease progression. There are only a few reports that suggest other bacterial pathogens elaborate factors that employ similar strategies. These include the oral streptococcal protein I/IIf that interacts with α 5 β 1 integrins [40] , and the YadA invasin of Yersinia pseudotuberculosis and the outer membrane protein, Opc of Nesseria meningitidis , both of which bind fibronectin to anchor to β 1 integrins resulting in bacterial uptake as well as IL-8 secretion [41] , [42] , [43] . Given that integrins preferentially localize to the basolateral surface of polarized endothelium [44] , we propose that these early molecular interactions of GBS with the BBB may alter cellular polarity as has been described for Helicobacter pylori [45] . It has also been demonstrated that GBS is capable of paracellular transit across an epithelial cell barrier where the bacterium co-localized with junctional protein complexes [46] . Whether these interactions act to disrupt tight junctional proteins and result in a non-polarized distribution of proteins on the BBB plasma membrane remains to be investigated. Our in vitro results were corroborated in vivo in a murine model of GBS haematogenous meningitis. Infection with the PilA-deficient mutant strain resulted in delayed mortality, decreased neutrophil infiltration and bacterial CNS dissemination and less expression of murine CXC chemokine KC. Histopathological analysis of the mice brains infected with WT GBS exhibited classical features of meningitis, such as thickening of the meninges, massive influx of inflammatory cells, specially neutrophils, and brain tissue damage. Also during the course of disease progression, significant differences in the bacterial load and KC levels between WT and Δ pilA mutant-infected animals were observed only in tissues that are typical sites of GBS infection such as brain and lung, whereas no difference was observed in other tissues including liver, kidney and spleen ( Supplementary Fig. S7 ). Thus, it is likely that other factors contribute to GBS CNS tropism. PilA-mediated virulence was also found to be dependent on neutrophil influx. Our results suggest that depletion of peripheral neutrophils conferred a survival benefit at later time points in GBS infection. Neutropenia was also accompanied by a decreased bacterial brain load and BBB permeability during infection. While some studies have demonstrated that the depletion of neutrophils was detrimental to the host during bacterial infection [47] , [48] , [49] , [50] , others have observed that PMN depletion prolonged host survival after infection [51] , [52] , [53] . Our findings demonstrate an association between leuckocyte trafficking and BBB permeability and increased GBS penetration of the CNS, suggesting that PMN-mediated damage of the BBB has a significant role in the pathogenesis of GBS meningitis. Overall, our findings suggest that GBS pili hijack host integrin machinery for inflammatory activation of brain endothelium and subsequent bacterial CNS entry. The resulting localized inflammation initiated by these early molecular events results in increased permeability of the BBB and facilitates bacterial passage from the blood stream to the immune privileged site of the CNS. To the best of our knowledge, this is the first report that describes the mechanistic and dual role of pili during CNS disease pathogenesis, as well the deleterious role of neutrophil infiltrate during GBS meningitis. Although currently there is no vaccine available for GBS infection, recent reports have identified GBS pili components, and PilA in particular as it is highly conserved between strains, as potential vaccine candidates [54] . Thus, our studies provide further mechanistic insight into the contribution of pili components to GBS disease pathogenesis. Bacterial strains Streptococcus agalactiae (GBS) serotype V strain NCTC 10/84 and its isogenic Δ pilA mutant that was created by in-frame allelic replacement with a chloramphenicol resistance cassette [8] were primarily used for the experiments. Mutations in the pilA gene in other GBS serotypes (serotype IA strain 515 and serotype III strain NEM316) were created by insertional duplication mutagenesis. Briefly, part of the pilA gene was amplified by PCR using the following set of primers; PilA(F): GTTTGTCGCAAATACCGCTTA and PilA(R): CATTACTCTCAACCTTAACTTG and cloned in pHY304. After transformation with respective recombinant plasmids insertional mutants were selected on Erythromycin selective plates. pilA gene deletion was confirmed by western blotting whole bacterial lysates using anti-PilA Ab. For complementation studies, full length pilA gene was amplified using the following sets of primers, KpnI–PilA(F): 5′-AGTCGGTACCATGAGAAAATA-3′; BglII–PilA(R): 5′-ATCGAGATCTTTAATCTTTTTC-3′ and cloned in pDCErm. Δ pilA mutant strain was transformed with the recombinant plasmid for generation of complemented strain. WT, Δ pilA mutants and complemented GBS strains were grown in Todd-Hewitt broth THB at 37 °C. Erythromycin at a concentration of 5 μg ml −1 was incorporated in the growth medium when required. Cell lines and infection assays The human brain microvascular endothelial cell line was kindly provided by Kwang Sik Kim (Johns Hopkins University) and cultured in RPMI1640 containing 10% FBS, 10% Nuserum and 1% nonessential amino acids [3] , [31] . hBMECs stably expressing shRNA targeting β 1 integrin (hBMEC Δβ 1 ) or cells expressing a control shRNA were generated by transfection (Santa Cruz Biotechnology). Knockdown of integrin β 1 was verified using standard flow cytometry assay (FACS; BD Biosciences). FAK–WT/hBMEC and FRNK/hBMEC cells are grown as reported [25] . Infection assays for microarray analysis, cytokine secretion, bacterial adherence and invasion were previously described [3] , [31] . Bacterial adherence and invasion was calculated as (recovered CFU/initial inoculum CFU)×100%. For inhibition studies, cells were pretreated for 30 min with indicated amounts of cytochalasin D, LY294002 and U0126, or 10 μg ml −1 of anti-integrin β 1 or anti-α 2 β 1 integrin Ab before incubation with bacteria. RT–PCR and ELISA RNA isolation, cDNA preparation and quantitative PCR was performed according to standard protocols. Primer sequences for IL-6, IL-8, CXCL1, CXCL2, CCL20, KC and β-actin and primer efficiencies are reported earlier [15] , [55] . Relative gene expression was calculated using the following equation: Relative gene expression=target gene efficiency×(CT control−CT sample)/efficiency for β-actin or GAPDH×(CT control−CT sample). Concentrations of IL-8, KC (R&D systems) or IL-1β and IL-6 (eBiosciences) in hBMEC supernatants or in mice tissue homogenates were determined by ELISA. Microarray analysis Microarray experiments were performed using Sentrix Human-8 Expression BeadChips (Illumina). Data were analysed using a statistical algorithm developed for high-density oligonucleotide arrays [56] . The microarray data has been deposited in the EMBL-EBI under accession code E-MTAB-765 . PilA–GST purification and generation of antiserum pilA gene from the genomic DNA of different GBS strains (serotype IA, III and V) was amplified using the following primers, SalI-PilA-F (5′-ATGCAGGTCGACAAGTACCGTACCGGAAAAT-3′), NotI-PilA-R (5′-ATGCAGCGGCCGCTTATCCTTTTGGTGGAATAT-3′) and cloned in pGEX4T-2 (GE HealthSciences). E. coli BL21(DE3) cells carrying pGEX–PilA were grown at 25 °C and protein expression was induced with 1 mM IPTG for 8 h. GST–PilA proteins were purified from the crude extracts using Glutathione–Sepharose (GE Healthsciences) column chromatography. Fractions collected were concentrated using Amicon Ultra centrifugal devices (Millipore) and buffer exchanged in PBS using PD10 columns (GE Healthsciences). Similarly purified GST served as a control protein. The proteins were made endotoxin-free using ToxinEraser Endotoxin Removal Kit (Genscript) and amount of endotoxin was quantitated using ToxinSensor Chromogenic LAL Endotoxin Assay Kit (Genscript). Anti-serum against PilA was generated by immunizing New Zealand white rabbits with PilA–(His) 6 protein preparation mixed with Freund's complete adjuvant (Pacific Immunology). The specificity of the anti-serum was determined by ELISA. Inhibitors and antibodies Following antibodies and inhibitors were used: rabbit anti-FAK, monoclonal anti-integrin β 1 and monoclonal anti-α 2 β 1 integrin (Millipore); monoclonal anti-GBS (Acris); monoclonal anti-FAK, FITC rat anti-mouse Ly6G and FITC rat IgG2a (BD Biosciences); anti-GST and goat polyclonal anti-Akt (Santa Cruz Biotechnology); monoclonal anti-FITC biotin conjugate and anti-laminin (Sigma); Alexa fluor 647 anti-mouse CD45 (BioLegend); anti-phospho p44/42 MAPK (pY204) and p44/42 MAPK rabbit Ab (Cell Signaling); rabbit polyclonal anti-phospho FAK (pY397) and rabbit polyclonal anti-phospho Akt (pS473) (Invitrogen); cytochalasin D, LY294002 (PI3K inhibitor), and U0126 (MEK1/2 inhibitor) (Sigma). Bacteria and PilA binding to collagen Bacterial binding to collagen was determined by crystal violet staining [57] . Stain bound to bacteria was released by addition of 20 mM citrate buffer, pH 4.3, and absorbance was measured at 595 nm. Binding of PilA–GST or GST to collagen was determined by ELISA [36] . ELISA plates coated with collagen I or BSA (2 μg per well) were treated with different concentration. of either PilA–GST or GST protein. After subsequent incubation with anti-PilA or anti-GST Ab and HRP-conjugated secondary Abs, chromophore was developed using 3,3′-, 5,5′-tetramethylbenzidine (Sigma) and the absorbance was measured at 450 nm. Cellular attachment of protein-coated latex beads Latex beads (1.1 μm in diameter, Sigma) were coated with PilA–GST or GST [58] proteins (1 mg ml −1 ) in coupling buffer (50 mM MES pH 6.1, 200 mM NaCl) at 4 °C for overnight. After washing, nonspecific sites were blocked with either 2% BSA or collagen. hBMEC monolayer was incubated with protein-coated latex beads at an approximate cell:bead ratio of 1:10 for 4 h. Confocal microscopy hBMECs treated with PilA protein or PilA-coated beads were fixed with 4% PFA and permeabilized with 0.1% triton X-100. PilA was stained with anti-PilA (1:1,000) Ab and Alexa Fluor 488 conjugated goat anti-rabbit Ab (Invitrogen). FAK was stained with anti-FAK Ab (1:1,000) followed by Cy5 conjugated rabbit anti-mouse Ab (Invitrogen). DNA was stained with To-Pro-3 iodide (Invitrogen). Coverslips were mounted on glass slides using Vectashiled (Vector labs) and visualized with a confocal laser scanning microscope (Leica Microsystems). Western blotting hBMEC were infected with WT GBS and Δ pilA mutant for different time points and lysed using RIPA buffer (Thermo Scientific) containing 2 mM Na 3 VO 4 , 100 mM NaF, 10 mM sodium pyrophosphate, 1 mM PMSF and protease inhibitor cocktail (Calbiochem). Cell lysates (40 μg) were probed with antibodies against phosphorylated and non-phosphorylated forms of FAK, Akt and Erk1/2 (all Abs at 1:1,000). In vivo neutrophil chemotaxis All animal experiments were approved by the Committee on the use and care of animals at San Diego State University (SDSU) protocol APF 10-08-024D and performed using accepted veterinary standards. Neutrophil recruitment was determined using a cutaneous in vivo neutrophil chemotaxis assay [15] , [55] . For determining signalling pathways resulting in neutrophil chemotaxis, 2 h before bacterial injection mice were injected subcutaneously with 1 mg kg −1 of U0126, LY294002 or DMSO. To assess PMN recruitment directly in the CNS, 5-day-old pups (C57BL/6, n =4 per group) were infected intracranially [59] with 1–3×10 5 CFU (25 μl) of either WT GBS or Δ pilA mutant. Following sacrifice, 8–10 h post infection, paraffin embedded brain sections were immunostained with FITC rat anti-mouse Ly6G (1:50) or stained with hematoxylin and eosin (H&E). Mouse model of haematogenous meningitis 8-week-old male CD-1 mice were injected intravenously with 6–7×10 7 CFU of WT GBS or isogenic Δ pilA mutant. At different time points after injection (24, 48 and 72 h), mice were euthanized and blood, brain and various other tissues such as lungs, spleen, liver and kidney were collected. One half of brain was fixed in 4% PFA for histopathological analysis. Of remaining brain tissue, ~30 mg was processed for RNA extraction. The remaining brain tissues as well as other tissues were homogenized in PBS and the homogenates were either plated on THA plates for enumeration of bacterial colonies or used for quantitation of chemokine KC by ELISA. Peripheral polymorphoneutrophil depletion PMN depletion was induced by the intraperitoneal administration of 50 μg of RB6–8C5 monoclonal Ab (BD Biosciences) to 6–8 weeks old CD-1 male mice 24 h before bacterial injection. Control mice received equivalent amount of isotype control Ab, rat IgG 2b . The extent of PMN depletion was determined by staining total blood leukocytes with with Alexa Fluor 647-labelled anti-CD45 and FITC-labelled anti-Ly6G antibodies (both at 1:500) and performing FACS at 24 and 48 h following injection of RB6–8C5 or IgG 2b . BBB permeability measurement BBB permeability was determined by EB vascular permeability as well as by leakage of FITC-albumin [28] , [29] . 1 h before ethuanization, 100 μl of 2% EB was injected i.v.. After sacrifice, mice brains were homogenized in PBS, proteins were precipitated by 60% trichloroacetic acid, and concentration of EB in the supernatants was determined by measuring absorbance at 610 nm. EB dye permeability is expressed as μg of EB per g of brain tissue against a standard curve. Alternatively, 30 min before sacrifice, mice were i.v. injected with 10 ml kg −1 of FITC-albumin, and brains were subsequently analysed by immunohistochemistry. Immunohistochemistry GBS was detected in brain sections by staining with anti-GBS Ab (1:20) and visualized using the Mouse on Mouse kit (Vector labs) containing a biotinylated anti-mouse IgG in conjunction with streptavidin-HRP. GBS was also detected by staining brain sections with anti-mouse secondary Ab conjugated to AlexaFluor 488. Blood vessels were labelled with Anti-laminin (1:50), nuclei with To-Pro, and the samples were viewed on a confocal microscope. Extravasation of FITC–albumin in the brains of mice was detected using an anti-FITC biotin conjugate (1:400) and visualized by streptavidin conjugated to Alexa Fluor 488. Statistical analysis Graphpad Prism version 4.03 was used for statistical analysis. Statistical significance was accepted at P <0.05. Acccession codes: The microarray data have been deposited in the EMBL nucleotide sequence database under accession code E-MTAB-765 . How to cite this article: Banerjee, A. et al . Bacterial Pili exploit integrin machinery to promote immune activation and efficient blood-brain barrier penetration. Nat. Commun. 2:462 doi: 10.1038/ncomms1474 (2011).